A role for DNA polymerase θ in the timing of DNA replication Although DNA polymerase θ (Pol θ) is known to carry out translesion synthesis and has been implicated in DNA repair, its physiological function under normal growth conditions remains unclear. Here we present evidence that Pol θ plays a role in determining the timing of replication in human cells. We find that Pol θ binds to chromatin during early G1, interacts with the Orc2 and Orc4 components of the Origin recognition complex and that the association of Mcm proteins with chromatin is enhanced in G1 when Pol θ is downregulated. Pol θ-depleted cells exhibit a normal density of activated origins in S phase, but early-to-late and late-to-early shifts are observed at a number of replication domains. Pol θ overexpression, on the other hand, causes delayed replication. Our results therefore suggest that Pol θ functions during the earliest steps of DNA replication and influences the timing of replication initiation. Human DNA polymerase θ (Pol θ) is a 290-kDa protein that comprises a carboxy-terminal A-family polymerase domain, which performs template-dependent and -independent DNA synthesis in vitro [1] , [2] , a large central domain of unknown function, and an amino-terminal domain that shares sequence similarity to known helicases, although no helicase activity has thus far been demonstrated [2] . Pol θ also exhibits deoxyribophosphodiesterase activity [3] and ATPase activity in the presence of single-stranded DNA [2] . The recombinant enzyme lacks the 3′→5′ exonuclease activity that is a common feature of low fidelity DNA polymerases and generates single base substitutions at an average rate comparable to the inaccurate Y family of DNA polymerases [2] , [4] , [5] . However, an active fraction of Pol θ purified from HeLa cells was shown to be capable of high fidelity of DNA polymerization [6] . This suggests that the enzyme may be accurate in a physiological context, perhaps through cooperation with proofreading co-factors. In spite of the intensive work aimed at understanding the cellular function(s) of this polymerase carried out over the past decade, a clear picture has yet to emerge as mostly species and cell type-specific functions have been reported. For example, studies performed in mice have suggested a role for Pol θ in somatic hypermutation of immunoglobulin genes [7] , [8] , [9] , but growing evidence indicate that such a function may be minor [10] . Pol θ has also been proposed to function in DNA repair. Indeed, this enzyme acts as a backup DNA polymerase during base excision repair in chicken DT40 cells [11] and nematodes [12] , but this functional observation has not been clearly demonstrated in mammals [13] , [14] , [15] . Studies in Drosophila have also suggested a role for Pol θ in the repair of double-stranded breaks through the synthesis of DNA during alternative microhomology-mediated end joining [16] , [17] . This potential DNA repair function could explain why mouse Pol θ-deficient bone marrow stromal cells and human Pol θ-depleted tumours exhibit increased sensitivity to ionizing radiation [13] , [14] . This role in the defense against ionizing radiation-induced DNA damage might also be due to the ability of the polymerase to perform translesion synthesis (TLS) past abasic sites and thymine glycol lesions, which are major products of reactive oxygen species-induced DNA damage and strong blockers to most other A-family as well as B-family replicative DNA polymerases [18] , [19] . The polymerase domain of Pol θ seems to be sufficient for this process, which relies on three insertion loops not present in other A-family DNA polymerases [18] . Moreover, Pol θ has the rare ability to catalyse both the insertion and the extension steps necessary to bypass the DNA lesion [19] , [20] , [21] . Nevertheless, a clear understanding of Pol θ physiological function and mechanism of action, especially under normal growth conditions, is still lacking. By conducting large-scale studies of the expression of DNA replication factors in patients with colon, breast and lung cancer, we recently uncovered major alterations in the expression pattern of POLQ , the gene encoding Pol θ, and discovered that excess POLQ correlates with genetic instability and poor prognosis [22] , [23] , [24] . This is, to our knowledge, the strongest link between a negative clinical outcome and the expression of a DNA polymerase [25] . The unique POLQ expression signature among replicative DNA polymerases and other specialized TLS and repair DNA polymerases—combined with the fact that Pol θ is the only human DNA polymerase that contains a helicase domain—prompted us to speculate that Pol θ might have an essential function in unstressed cells. To determine the role of Pol θ during normal DNA replication in human cells, we asked whether either loss or excess of Pol θ could affect the DNA replication programme under physiologic growth conditions. These experiments uncovered an unexpected requirement for Pol θ for proper minichromosome maintenance (Mcm) loading during G1 and the timing of DNA replication at a subset of domains during S phase. Association of Pol θ with chromatin in early G1 We first studied in detail Pol θ recruitment onto chromatin during the cell cycle by using unstressed human RKO cells under physiological growth conditions (5% oxygen concentration). Cells were synchronized in pro-metaphase with nocodozole, collected by mitotic shake-off, released into the cell cycle and then analysed at various times throughout M, G1 and S phases. We checked cell cycle progression and S phase entry by bromodeoxyuridine (BrdU) incorporation, propidium iodide staining and fluorescence-activated cell sorting analysis ( Fig. 1 , left panel). Cell extracts were then fractionated and chromatin fractions were subjected to immunoblotting ( Fig. 1 , right panel). Unexpectedly, detectable Pol θ was found in the chromatin fraction as cells exited mitosis. Its level in this fraction then increased greatly in early G1 and persisted until S phase. As G1 is the phase where the replication origins are set up and the pre-replication complexes (pre-RCs) formed [26] , [27] , we compared the timing of Pol θ recruitment with the kinetics of pre-RC assembly. As expected, Origin recognition complex subunit 2 (Orc2) and cell division control protein 6 (Cdc6) were associated with chromatin in mitosis and remained there as cells entered G1. Next, Cdt1 (Cdc10 protein-dependent transcript 1) was recruited, followed by the recruitment of Mcm helicases and the downregulation of Cdc6 (ref. 28 ). As also expected, when cells entered S phase the enzymes involved in DNA synthesis, including the replicative A-family DNA polymerases Pol α and Pol δ, were recruited and Cdt1 released. Strikingly, Pol θ was found to be recruited to chromatin just before Mcm. All of these observations were confirmed using the Cdk1 inhibitor RO-3306 as an alternative mode of cell synchronization ( Supplementary Fig. 1 ). Under these conditions, Pol θ was recruited to chromatin concomitantly with Mcm. These results appear to be the first evidence of a DNA polymerase being loaded onto chromatin in early G1 in the absence of external stress. 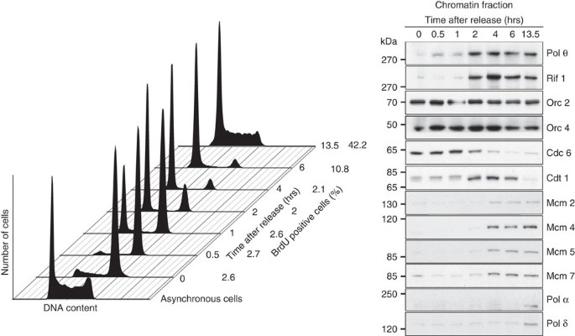Figure 1: Pol θ is recruited to chromatin in early G1 in human cells. Cells of the human RKO line were synchronized in mitosis by nocodazole treatment (0.1 μM, 20 h) and then released into fresh medium for the indicated times (0, 30 min, 1, 2, 4, 6 h and 13 h 30 min). Cell cycle progression was followed by fluorescence-activated cell sorting analysis after BrdU incorporation and propidium iodide staining (left panel). The recruitment of Pol θ onto chromatin through the cell cycle was analysed by western blotting after subcellular fractionation (right panel). The time course of chromatin binding for Rif1, the pre-replication complex and the replicative DNA polymerases α and δ were also checked (right panel). Equivalent cell number fractions were loaded. This figure is representative of three independent experiments. Figure 1: Pol θ is recruited to chromatin in early G1 in human cells. Cells of the human RKO line were synchronized in mitosis by nocodazole treatment (0.1 μM, 20 h) and then released into fresh medium for the indicated times (0, 30 min, 1, 2, 4, 6 h and 13 h 30 min). Cell cycle progression was followed by fluorescence-activated cell sorting analysis after BrdU incorporation and propidium iodide staining (left panel). The recruitment of Pol θ onto chromatin through the cell cycle was analysed by western blotting after subcellular fractionation (right panel). The time course of chromatin binding for Rif1, the pre-replication complex and the replicative DNA polymerases α and δ were also checked (right panel). Equivalent cell number fractions were loaded. This figure is representative of three independent experiments. Full size image Pol θ interacts with Orc2 and Orc4 Assembly of the pre-RC complex starts with the binding of Orc. This then serves as a platform for the loading of Cdc6, Cdt1 and Mcm2–7. Our observation that Pol θ associates with chromatin around the time of pre-RC formation in early G1 prompted us to analyse whether Pol θ may interact directly with the Orc platform. First, a Pol θ antibody was used to immunoprecipitate Pol θ from cell lysates. Orc2 and Orc4 antibodies were then used to test for the presence of Orc2 and Orc4 by western blotting ( Fig. 2a ). We identified Orc2 and Orc4 in Pol θ immunoprecipitates and these interactions were confirmed by performing immunoprecipitation with different Orc2 and Orc4 antibodies followed by western blot analysis of the immunoprecipitated Pol θ ( Fig. 2a ). To the best of our knowledge, Orc2 and Orc4 are the first identified proteins that can interact with Pol θ. These data suggest that Pol θ could bind to replication origins. 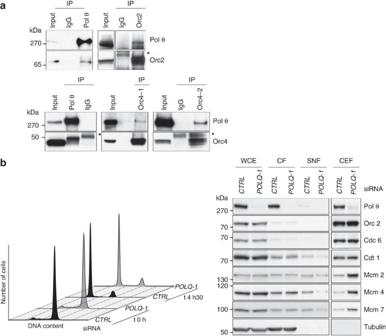Figure 2: Pol θ interacts with Orc2 and Orc4, and controls Mcm loading onto chromatin in G1. (a) Pol θ interacts with Orc2 and Orc4. RKO cell extracts were immunoprecipitated with Pol θ, Orc2, or Orc4 antibodies (Orc2-1, Orc4-1 and Orc4-2) and analysed by western blotting using anti-Pol θ, Orc2 or Orc4-2 antibodies; asterisk (*) corresponds to IgG. (b) Thirty hours after Control (CTRL) orPOLQ-1siRNA transfection, RKO cells were synchronized in G2/M with nocodazole (0.1 μM, 20 h), released into fresh medium, and then collected 270 min later in G1. Cell cycle analysis of mock- (CTRLsiRNA) and Pol θ- (POLQ-1siRNA)-depleted cells was performed by propidium iodide staining and fluorescence-activated cell sorting analysis (left panel). Cell fractionation was performed and processed for immunoblotting with the indicated antibodies (right panel). All blots are representative of three independent experiments. WCE, whole cell extract; CF, cytoplasmic fraction; SNF, soluble nuclear fraction; CEF, chromatin-enriched fraction. Orc2 and Tubulin serves as fractionation and loading controls. Uncropped blots shown in (a) are shown inSupplementary Fig. 8. Figure 2: Pol θ interacts with Orc2 and Orc4, and controls Mcm loading onto chromatin in G1. ( a ) Pol θ interacts with Orc2 and Orc4. RKO cell extracts were immunoprecipitated with Pol θ, Orc2, or Orc4 antibodies (Orc2-1, Orc4-1 and Orc4-2) and analysed by western blotting using anti-Pol θ, Orc2 or Orc4-2 antibodies; asterisk (*) corresponds to IgG. ( b ) Thirty hours after Control ( CTRL ) or POLQ-1 siRNA transfection, RKO cells were synchronized in G2/M with nocodazole (0.1 μM, 20 h), released into fresh medium, and then collected 270 min later in G1. Cell cycle analysis of mock- ( CTRL siRNA) and Pol θ- ( POLQ-1 siRNA)-depleted cells was performed by propidium iodide staining and fluorescence-activated cell sorting analysis (left panel). Cell fractionation was performed and processed for immunoblotting with the indicated antibodies (right panel). All blots are representative of three independent experiments. WCE, whole cell extract; CF, cytoplasmic fraction; SNF, soluble nuclear fraction; CEF, chromatin-enriched fraction. Orc2 and Tubulin serves as fractionation and loading controls. Uncropped blots shown in ( a ) are shown in Supplementary Fig. 8 . Full size image Pol θ regulates Mcm loading onto chromatin in G1 Our observations that Pol θ interacts with Orc2 and Orc4 prompted us to explore whether Pol θ is required for pre-RC formation. Therefore, we analysed pre-RC assembly in G1 in the absence of Pol θ ( Fig. 2b ). Small interfering RNA (siRNA)-mediated POLQ gene silencing was performed in RKO cells with a near-complete depletion of Pol θ ( Fig. 2b , right panel). Pol θ depletion did not affect cell cycle progression even after long-term downregulation ( Supplementary Fig. 2A ) and did not trigger the activation of the DNA damage signalling ( Supplementary Fig. 2B ). Mock and Pol θ-depleted cells were synchronized in G2/M with nocodazole and then released into fresh medium and collected in G1 270 min after release ( Fig. 2b , left panel). Cell extracts were fractionated and immunoblotting of the resulting fractions revealed that when Pol θ was downregulated the binding of Orc2, Cdc6 and Cdt1 to chromatin remained unchanged ( Fig. 2b , right panel). In contrast, the association of Mcm2, Mcm4 and Mcm7 with chromatin was significantly increased in the absence of Pol θ. These observations were confirmed in a separate POLQ siRNA experiment where cell synchronization was achieved using the Cdk1 inhibitor RO-3306 ( Supplementary Fig. 3 , right panel). Mcm accumulation was not due to a cycle effect, as Pol θ depletion did not lead to a significant modification of cell cycle progression ( Fig. 2b , left panel, and Supplementary Fig. 3 , left panel). Therefore, collectively these results show that Pol θ plays an important role in controlling the association of Mcm with chromatin in G1. As the Mcm complexes are known to be initially recruited and enriched at replication origins during G1 and as Pol θ interacts with Orc2 and Orc4, this suggests that Pol θ contributes to the proper formation of pre-RC complexes directly at replication origins. Pol θ does not control origin density We next hypothesized that the increased Mcm loading seen in G1 in Pol θ-deficient cells may lead to an increased number of origins, including active origins. To test this, we quantified the density of active origins using single molecules analysis by DNA combing, after sequential pulse-labelling of control, and Pol θ-depleted cells with the nucleotide analogues IdU and CldU [29] . We first measured the inter-origin distances (IODs) at the genome-wide level, which revealed the number of active origins within replication domains. We did not observe a significant change in IODs in Pol θ-depleted cells relative to control cells ( Fig. 3a ). We then monitored global fork density, which reflects the number of active origins both within and between different replication domains. Again, we found that the global fork density, measured as the number of forks divided by the total length of DNA fibres and normalized by the percentage of cells in S phase, remained unchanged following Pol θ downregulation (~ 0.9 fork per Mb) ( Fig. 3b ). As a positive control, we verified that upon replication stress (low doses of Hydoxyurea), RKO cells showed inhibition of distant origins, as revealed by a decreased fork density ( Supplementary Fig. 4 ). From these experiments we concluded that the increased Mcm loading in G1 in Pol θ-depleted cells did not result in increased origin firing during S phase, suggesting that the loss of Pol θ did not lead to the formation of additional pre-RCs. This conclusion is supported by our observations that loading of the pre-RC proteins Cdc6 and Cdt1 was not significantly increased following Pol θ depletion ( Fig. 2b , right panel). 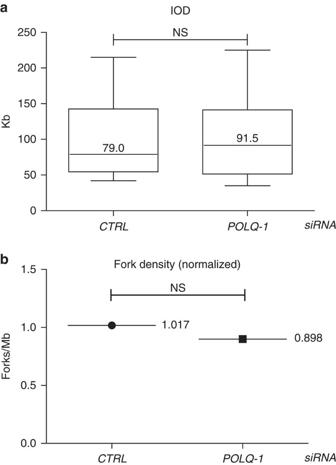Figure 3: Pol θ depletion does not affect the fork density and the inter-origin distances. DNA replication was monitored on single molecules spread by DNA combing in mock- (CTRL siRNA) and Pol θ- (POLQ-1 siRNA) depleted cells after sequential pulse-labelling with IdU and CldU. Inter-origin distances (a) and fork density (b) were analysed. The non-parametric test of Mann–Whitney was applied to compare data sets from control and Pol θ-depleted cells. Figure 3: Pol θ depletion does not affect the fork density and the inter-origin distances. DNA replication was monitored on single molecules spread by DNA combing in mock- (CTRL siRNA) and Pol θ- (POLQ-1 siRNA) depleted cells after sequential pulse-labelling with IdU and CldU. Inter-origin distances ( a ) and fork density ( b ) were analysed. The non-parametric test of Mann–Whitney was applied to compare data sets from control and Pol θ-depleted cells. Full size image Pol θ depletion affects the replication timing As the increased level of Mcm accumulation onto chromatin in the absence of Pol θ did not result in a change in origin density, we investigated whether the timing of origin activity could be affected in Pol θ-depleted cells. Activation of replication origins is controlled by a specific timing programme established in early G1 phase at the so called ‘timing decision point’ (TDP) [30] , [31] . Replication timing is a highly stable cell type-specific process whose mechanistic basis remains poorly understood in vertebrates [32] , [33] , [34] . The data presented in Fig. 1 show that the timing of the association of Pol θ with chromatin is close to that of the TDP. Moreover, it coincides with the loading of Rap-interacting-factor-1 (Rif1) ( Fig. 1 , right panel), recently discovered as the first molecular regulator of replication timing [32] , [34] , [35] . We therefore speculated that Pol θ could contribute to the determination of the replication timing profile. This issue was addressed by analysing the timing of replication domains in control and Pol θ-depleted cells ( Fig. 4a ) at a genome-wide level. Cells were pulse-labelled with BrdU and separated into early and late S-phase fractions by flow cytometry as previously described [31] , [36] (see Methods). To examine replication timing, a CGH algorithm developed by the AGILENT company was used. It generates segments corresponding to both the early replication domain when the log-ratio is positive and conversely the late replication domain when the log-ratio is negative ( Fig. 4b and Supplementary Fig. 5 ). The loss of Pol θ resulted in a modification in replication timing of ~5% of the human genome with an equivalent number of early-to-late (EtoL) and late-to-early (LtoE) switches (a global analysis is shown in Supplementary Fig. 5 ; one example from two independent experiments is presented in Fig. 4b , with black and grey arrows indicating EtoL and LtoE changes, respectively). These results clearly show that the replication timing of a subset of domains is modified following Pol θ depletion. The observation that Pol θ and Rif1 showed similar profiles of association onto chromatin after mitosis and in G1 ( Fig. 1 and Supplementary Fig. 1A ) further supports the idea that Pol θ contributes towards setting up the TDP. Importantly, Pol θ depletion affected neither the global level of Rif1 nor its recruitment onto chromatin in G1 ( Fig. 4a and Supplementary Fig. 6A,B ). Furthermore, in contrast to Pol θ-depleted cells, Rif-1-depleted cells display no change in pre-RC formation, longer IOD and changes in replication timing that occur in middle S-phase domains [34] . Collectively, these observations suggest that similar to Rif1, Pol θ plays a role in establishing the TDP but that the mechanisms of action of Pol θ and Rif1, as well as their targeted sub-domains, are distinct. 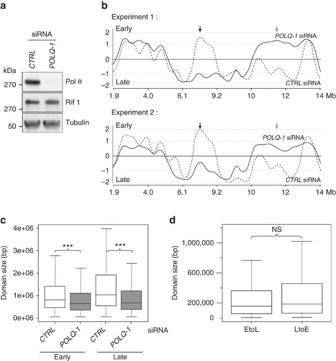Figure 4: Pol θ depletion modifies the temporal replication programme. (a) Western blot analysis with the indicated antibodies of whole-cell extracts from mock- (CTRLsiRNA) and Pol θ- (POLQ-1siRNA) depleted RKO cells used for the replication timing experiments shown inbandSupplementary Fig. 2. (b) The replication timing was analysed 24 h after transfection withCTRLorPOLQ-1siRNA. Shown are the microarray profiles of the timing of replication on chromosome 6: 1 997 799–14 527 487 (12.5 Mb, hg18) from two independent experiments. Black lines representPOLQ-1siRNA and dotted lines represent control (CTRL) siRNA. Arrows indicate examples of changes in replication timing. Black arrows: early to late (EtoL); grey arrows: LATE TO Early (LtoE). The size of the replication domains (c) and the size of the domains where replication timing was changed (d) were analysed. The thick line represents the median, the limit of the box corresponds to the 0.25 to 0.75 quartiles with whiskers extending to the maximum value of 1.5 times the interquartile range; Early: early domains, Late: late domains, EtoL: early-to-late, LtoE: late-to-early; ***P-value<0.001. Data are representative of two independent experiments of microarrays for each siRNA experiments and thus generate more than 700 domains for each categories. Statistical significance was performed with Student’st-test from the R package. The characteristic of thet-test incis:t=6.0954, df=1750.042,P-value=1.34e−09, indicating here the significance of the test. Uncropped blots are shown inSupplementary Fig. 8. Figure 4: Pol θ depletion modifies the temporal replication programme. ( a ) Western blot analysis with the indicated antibodies of whole-cell extracts from mock- ( CTRL siRNA) and Pol θ- ( POLQ-1 siRNA) depleted RKO cells used for the replication timing experiments shown in b and Supplementary Fig. 2 . ( b ) The replication timing was analysed 24 h after transfection with CTRL or POLQ-1 siRNA. Shown are the microarray profiles of the timing of replication on chromosome 6: 1 997 799–14 527 487 (12.5 Mb, hg18) from two independent experiments. Black lines represent POLQ-1 siRNA and dotted lines represent control ( CTRL ) siRNA. Arrows indicate examples of changes in replication timing. Black arrows: early to late (EtoL); grey arrows: LATE TO Early (LtoE). The size of the replication domains ( c ) and the size of the domains where replication timing was changed ( d ) were analysed. The thick line represents the median, the limit of the box corresponds to the 0.25 to 0.75 quartiles with whiskers extending to the maximum value of 1.5 times the interquartile range; Early: early domains, Late: late domains, EtoL: early-to-late, LtoE: late-to-early; *** P -value<0.001. Data are representative of two independent experiments of microarrays for each siRNA experiments and thus generate more than 700 domains for each categories. Statistical significance was performed with Student’s t -test from the R package. The characteristic of the t -test in c is: t =6.0954, df=1750.042, P -value=1.34e−09, indicating here the significance of the test. Uncropped blots are shown in Supplementary Fig. 8 . Full size image For both control and Pol θ-depleted cells, the range of the sizes of the replication domains varied from ~10 kb to 1.5 Mb, with several domains larger than 2 Mb (up to 8 Mb), in close agreement with previous reports in human and mouse cell lines [31] ( Fig. 4c ). Moreover, late domains were always significantly larger than early domains for the control cells ( Fig. 4c , P -value=1.418e−10), as previously observed in mammalian cell lines [31] . This could be due to the acceleration of replication forks or alternatively to increased activation of stochastic origins in late S-phase, as has already been suggested [37] . Strikingly, in contrast to control cells the sizes of the late and early domains were not significantly different in the Pol θ-depleted cells ( Fig. 4c ) and were both significantly reduced compared with control cells (early CTRL siRNA/early POLQ siRNA: P -value=1.34e−09; late CTRL siRNA/late POLQ siRNA: P -value<2.2e−16). We observed 240 EtoL regions (early in control cells to late in Pol θ-depleted cells) corresponding to a delay of the replication timing in Pol θ-depleted cells in comparison with the control cells, and 244 LtoE regions (late in control cells to early in Pol θ-depleted cells). These regions where the timing is modified display an equivalent average size ( Fig. 4d ) and show similar molecular characteristics that have been observed during cell differentiation by Hiratani et al . [31] Characterization of the modified domains The domains in which replication timing was changed in the absence of Pol θ were then characterized. Mammalian chromosomes are organized in alternative AT- and GC-rich sequences that are rich and poor in Line-1 transposable elements, respectively [38] . Several studies have previously reported a strong positive correlation between Line 1 content, GC content, gene density and early replication [33] , [39] . Such a correlation was also detectable in RKO control cells ( Fig. 5a–c ). Interestingly, the loss of Pol θ induced EtoL and LtoE domains that presented an intermediate Line-1 content ( Fig. 5a ), gene density ( Fig. 5b ) and GC content ( Fig. 5c ), similar to what was observed during cell differentiation by Gilbert and colleagues [31] . Recently, it was demonstrated that G-quadruplex (G4), a G-rich DNA sequence that can form a four stranded structure, is associated with DNA replication origins [40] , [41] . Despite the absence of consensus sequences that could define replication origins, the presence of these G4 motifs may play a critical role in their localization and/or activation. As the probability of containing G4 motifs is increased in GC-rich sequences, the measures of G4 density were normalized with the GC content. As has been previously shown in different human and mouse cell lines [40] , [41] , we confirmed here that early replicating domains are enriched in G4 motifs in RKO control cells ( Fig. 5d ). Next, we monitored G4 density in the domains where replication timing had been changed following Pol θ depletion. As G4 motifs strongly correlate with replication origins, measuring G4 density allows an indirect assessment of the number of potential replication origins in E, EtoL, LtoE and L domains. As for Line-1 content, gene density and GC content, EtoL and LtoE domains showed an intermediate G4 content ( Fig. 5d ), reflecting an intermediate level of potential origins. The characteristics of all the domains EtoL and LtoE are presented in Supplementary Tables 1 and 2 , respectively. 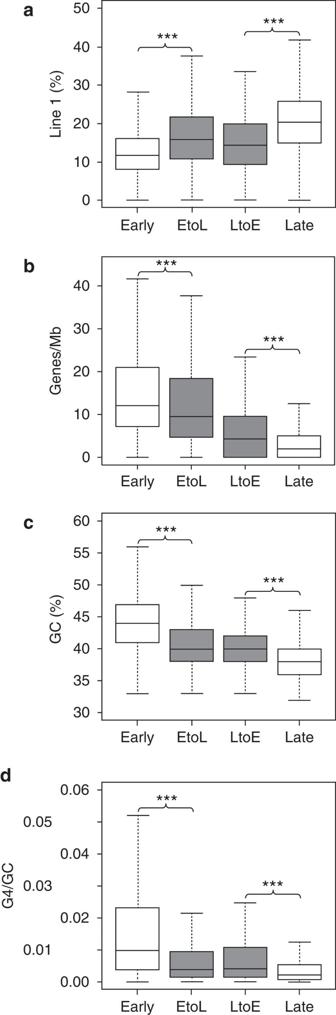Figure 5: Characterization of the domains in which replication timing was changed following Pol θ depletion. Analysis of Line-1 content (a), gene density (b), GC content (c) and G4/GC content (d) in Early domains, early-to-late domains (EtoL), late-to-early domains (LtoE) and late domains in Pol θ-depleted cells. The statistical significance was performed with Student’st-test from the R package. The thick line represents the median, the limit of the boxes corresponds to the 0.25 to 0.75 quartiles with whiskers extending to the maximum value of 1.5 times the interquartile range. ***P-value<0.001. Data are representative of two independent microarrays experiments for each siRNA, generating more than 700 domains for each categories. Thet-test characteristics aret=3.3644, df=298.512,P-value=8.6e−4 forb;t=6.78, df=314.213,P-value=5.9e−17 forc; andt=5.0732, df=557.542,P-value=5.335e−07 ford, indicating the significance of the test. Figure 5: Characterization of the domains in which replication timing was changed following Pol θ depletion. Analysis of Line-1 content ( a ), gene density ( b ), GC content ( c ) and G4/GC content ( d ) in Early domains, early-to-late domains (EtoL), late-to-early domains (LtoE) and late domains in Pol θ-depleted cells. The statistical significance was performed with Student’s t -test from the R package. The thick line represents the median, the limit of the boxes corresponds to the 0.25 to 0.75 quartiles with whiskers extending to the maximum value of 1.5 times the interquartile range. *** P -value<0.001. Data are representative of two independent microarrays experiments for each siRNA, generating more than 700 domains for each categories. The t -test characteristics are t =3.3644, df=298.512, P -value=8.6e−4 for b ; t =6.78, df=314.213, P -value=5.9e−17 for c ; and t =5.0732, df=557.542, P -value=5.335e−07 for d , indicating the significance of the test. Full size image These analyses strengthen the notion that regions where replication timing can change possess specific genomic signatures, as Gilbert and colleagues [31] have previously proposed, and further support the model that Pol θ is a regulator of replication timing of particular regions of the human genome. Excess Pol θ delays replication timing To obtain more insight into the mechanism by which Pol θ contributes to replication timing, we analysed the impact of the excess of Pol θ on replication timing at a genome-wide level. We generated human cells that stably overexpress Pol θ compared with the endogenous Pol θ level of the isogenic control [23] ( Fig. 6a ) and examined replication timing as described above. Excess Pol θ resulted mostly in a delayed timing of multiple domains (a global analysis is shown in Supplementary Fig. 7 ; two examples are presented in Fig. 6b ). It is important to note that as seen with Pol θ depletion, overexpression of Pol θ had no impact on the global level of Rif1 ( Fig. 6a ). These results clearly show that excess Pol θ delays the replication timing of a subset of domains. 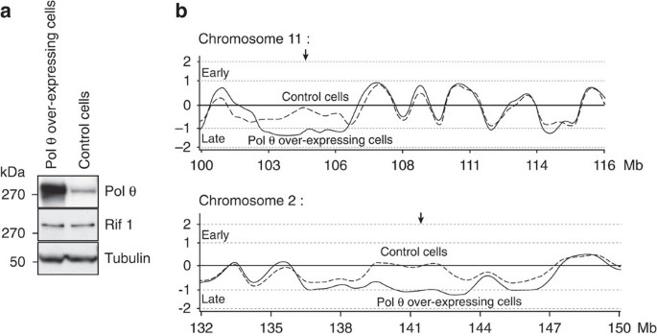Figure 6: Excess Pol θ leads to a delayed replication of several replicating domains. (a) Western blot analysis with the indicated antibodies of whole-cell extracts from control and overexpressing MRC5 cells used for the replication timing experiments shown inbandSupplementary Fig. 4. (b) Two examples of microarray profiles of the timing of replication on chromosomes 11 and 2 in Pol θ-overexpressing cells and isogenic control cells. Uncropped blots are shown inSupplementary Fig. 8. Figure 6: Excess Pol θ leads to a delayed replication of several replicating domains. ( a ) Western blot analysis with the indicated antibodies of whole-cell extracts from control and overexpressing MRC5 cells used for the replication timing experiments shown in b and Supplementary Fig. 4 . ( b ) Two examples of microarray profiles of the timing of replication on chromosomes 11 and 2 in Pol θ-overexpressing cells and isogenic control cells. Uncropped blots are shown in Supplementary Fig. 8 . Full size image Shortly after mitosis, daughter cells organize their genomes into large replication domains containing multiple replication initiation sites that are activated simultaneously. The organization of replication domains occurs during the G1 phase of the cell cycle at the TDP. Although orderly progression of DNA replication is important to ensure stable genetic and epigenetic inheritance, the mechanisms underlying the timing programme of replication have yet to be fully elucidated. Here we have identified a novel actor of the human DNA replication timing programme, Pol θ, an enzyme classified thus far as a specialized repair A-family DNA polymerase [2] , [42] . We first presented evidence that the timing of association of Pol θ with chromatin appears to be similar to that of pre-RC formation and is concomitant with Mcm loading. Moreover, we show that Pol θ interacts with Orc2 and Orc4, subunits of the Orc platform for the loading of pre-RC components. Finally, Pol θ-depleted cells demonstrated multiple abnormalities: increased Mcm loading onto chromatin in G1 and genome-wide changes in replication timing of a subset of domains with no modification of origin density. All these data are consistent with the hypothesis that Pol θ plays a role at or near the TDP by regulating the number of Mcm molecules at individual pre-RCs. Interestingly, computational analysis of replication timing has previously indicated that replication timing can be regulated by the number of Mcm molecules bound to the origin and the chromatin context [43] . This model predicts that origins with more loaded Mcm have a higher probability of firing and thus an earlier average replication time [43] . We propose the following model to explain our results: when Pol θ is expressed, it could bind to the Orc at a subset of individual late origins in G1 and inhibits the recruitment of excess Mcm to avoid early replication timing of these late origins. When Pol θ is depleted, increased Mcm loading at these individual late origins could be facilitated, possibly via enhanced interaction with Orc, resulting in the observed LtoE switch. The abnormal recruitment of activating limiting factors to these advanced late origins could reduce the full availability of these factors locally at some early origins, explaining why the activation of some early origins are delayed (EtoL). When Pol θ is overexpressed, it could bind also early–middle origins through Orc interaction and consequently delay their activation. We therefore propose that in human cells Pol θ establishes some late S-phase replication domains that are restrained from being activated at early S phase. The discovery that Pol θ contributes to the regulation of DNA replication timing in human cells is of particular interest, as the regulation of this programme is extremely robust. In vertebrates, only the loss of Rif1 has been shown thus far to affect replication timing of a subset of domains [32] , [34] . Rif1 was originally discovered as a telomere-binding protein in yeast [44] and a double-strand break response factor in mammals [45] , and has previously been shown to regulate the timing of replication in yeast [35] . Importantly, our data suggest that although Pol θ and Rif1 display similar binding kinetics to chromatin at TDP when cells exit mitosis, their roles in controlling replication timing seem to be different. Indeed, in contrast to Pol θ, Rif1 seems to establish mid S-phase replication domains that are restrained from being activated at early S phase, without any impact on pre-RC formation [32] , [34] . Moreover, Pol θ depletion affects neither the global level of Rif1 nor its recruitment to chromatin in G1. Pol θ is encoded by the POLQ gene that is present in plants and multicellular eukaryotes but not yeast or other fungi [46] . Although mammalian Pol θ is often best known for its proposed role in repair of genome damage, it appears that there are important functional differences between species and cell types. Moreover, very little of its physiological function in unstressed cells has been thoroughly investigated. The TEBICHI (TEB) gene, encoding a Pol θ-like protein found in Arabidopsis thaliana , is required for normal plant development in the absence of external stress [47] , [48] . Both the POLQ knockout mouse [49] and the chaos1 (chromosome aberration occurring spontaneously 1) mouse that possesses a mutant allele of POLQ [50] show increased manifestations of spontaneous genetic instability, with enhanced formation of micronuclei. Interestingly, in the same screen that identified the chaos1 allele of POLQ , a second mutant called chaos3 exhibited a similar phenotype of increased micronuclei [51] . Chaos3 was identified as a hypomorphic allele of Mcm4, a component of the hexameric Mcm helicase complex. Our data also provide new information on the role of Pol θ during the cell cycle in unstressed cells, and extend the function of Pol θ to include normal DNA replication, strengthening the concept that TLS or repair synthesis after external stress might not be the sole function assigned to non-replicative DNA polymerases. We recently showed that this is the case for both Pol η, which is required for the stability of common fragile sites during unperturbed S-phase [52] , [53] , and Pol κ, which functions at stalled forks in unstressed cells to ensure high cell viability and genomic stability [54] . This novel Pol θ function may be particularly important within the context of cancer, as high POLQ expression is strongly associated with poor clinical outcome of patients with colon, breast and lung cancers [22] , [23] , [24] , [55] , [56] . Abnormal temporal control of replication, recently demonstrated in several haematologic malignancies, has been proposed to represent a common mechanism responsible for genomic instability found in cancer cells [57] ; therefore, Pol θ overexpression may be of cardinal importance in defining the modified temporal replication programme in cancer cells and may constitute a driving force for chromosomal instability [58] , [59] , [60] . Cell line and culture conditions The human RKO cell line was purchased from ATCC and grown in DMEM with GlutaMAX I, high-glucose, sodium pyruvate (Gibco, Life Technologies, Paisley, UK), supplemented with 10% fetal bovine serum (Lonza, Basel, CH), penicillin (100 U ml −1 ) and streptomycin (100 μg ml −1 ) (Gibco) at 37 °C, 5% CO 2 and 5% O 2 (standard culture conditions). The design and construction of the POLQ expression vector as well as the overexpressing Pol θ cells (Q3) and their isogenic controls (Ctrl2) were previously described [23] . They were grown in Modified Eagle’s Medium-α with GlutaMAX I, high-glucose, sodium pyruvate (Gibco, Life Technologies) supplemented with 10% fetal bovine serum (Lonza), hygromycin B (50 μg ml −1 ), penicillin (100 U ml −1 ) and streptomycin (100 μg ml −1 ) (Gibco) at 37 °C, 5% CO 2 and 5% O 2 . Transfection of siRNA RKO cells were transfected with siRNA targeting either POLQ or Luciferase (CTRL). POLQ-1 is an siRNA ON-TARGET plus smart pool of four POLQ siRNA from Dharmacon (Thermo Fisher Scientific, Waltham, USA): 5′-CCUUAAGACUGUAGGUACU-3′, 5′-ACACAGUAGGCGAGAGUAU-3′, 5′-CGACUAAGAUAGAUCAUUU-3′ and 5′-CAAACAACCCUUAUCGUAAA-3′. POLQ-2 is an siRNA ON-TARGET plus smart pool of four POLQ siRNA from Dharmacon: 5′-UCAGAGGGAUGGAGCUAAU-3′, 5′-GAGAUUACCCUUUCACCUA-3′, 5′-AAUUUUACAGUACGGAAA-3′ and 5′-UGAUAGAUUAGCCUAGUA-3′. For Luciferase (CTRL) , 5′-CGUACGCGGAAUACUUCGAdTdT-3′ (Sigma-Aldrich, Saint-Louis, USA) was used. siRNAs were used at a final concentration of 50 nM, using the Lipofectamine 2000 transfection reagent (Invitrogen, Carlsbad, USA) following the manufacturer’s suggestions. The transfection medium was replaced 8 h later by complete medium. Cell synchronization Cells were synchronized in mitosis by nocodazole (0.1 μM, Sigma-Aldrich) for 20 h. Next, cells were collected by mitotic shake-off, washed twice in warm complete medium and released into the cell cycle under standard culture conditions. At the indicated times, cells were collected for subcellular fractionation and BrdU incorporation assay. When cells were transfected with POLQ-1 or CTRL siRNA, nocodazole was added to the medium 30 h later. For cell synchronization in G2/M with RO-3306, cells were incubated for 20 h with RO-3306 (9 μM, Sigma-Aldrich), then released after 2 washes in warm complete medium. Thirty minutes later, mitotic cells were collected by mitotic shake-off and released into the cell cycle under standard culture conditions. At the indicated times, cells were collected for subcellular fractionation and a BrdU incorporation assay. As a control, asynchronous cells were incubated with dimethyl sulphoxide (Sigma-Aldrich) instead of RO-3306. When cells were transfected with POLQ-2 or CTRL siRNA, RO-3306 was added 26 h after transfection. BrdU incorporation assay Cells were pulse-labelled with 10 μM BrdU (Sigma-Aldrich) for 15 min then collected by trypsinization and fixed in 70% ethanol overnight at −20 °C. After washing with PBS–BSA 0.5% (Sigma-Aldrich), DNA was denatured for 20 min with 2 N HCl treatment (Normapur, VWR, Lutterworth, UK) at room temperature (RT). Cells were washed in PBS–BSA 0.5%, incubated with sodium tetraborate (0.1 M, pH 8.5) for 2 min at RT, washed and then incubated with a mouse anti-BrdU fluorescein isothiocyanate antibody (1:25, Becton Dickinson) in PBS–BSA 0.5%, Tween20 0.5%, for 1 h at RT. After washing, Alexa Fluor 488 goat anti-mouse IgG (1:50, Invitrogen) was added in PBS–BSA 0.5%, Tween20 0.5% for 30 min at RT. Finally, after washing in PBS–BSA 0.5%, then in PBS, cells were resuspended in PBS with propidium iodide (25 μg ml −1 , Sigma-Aldrich) and RNase A (100 μg ml −1 , Thermo Fisher Scientific). After 20 min of incubation at RT, cell cycle analysis was carried out by flow cytometry with a FACScalibur cytometer (Becton Dickinson). Whole-cell extracts Cells were resuspended in lysis buffer (Tris-HCl: 50 mM, pH 7.5, NaCl 250 mM, EDTA 1 mM, Triton X-100 0.1%, with protease inhibitors) for 30 min on ice. After centrifugation at 15,000 rcf, for 20 min at 4 °C, the supernatant was collected. Laemmli buffer was added and the mixture boiled for 3 min. Cell fractionation Subcellular fractionation was performed as described previously [61] . Briefly, cells were lysed in Buffer A (Hepes 10 mM pH 7.9, KCl 10 mM, MgCl 2 1.5 mM, sucrose 0.34 M, Glycerol 10%, dithiothreitol (DTT) 1 mM, Halt protease and phosphatase inhibitor cocktail from Thermo Fisher Scientific) complemented with Triton X-100 0.1% for 5 min on ice. After centrifugation at 1,500 rcf, 5 min, 4 °C, the supernatant was clarified by high-speed centrifugation (18,000 rcf, 4 °C, 15 min) to obtain the cytoplasmic fraction. The pellet was washed once with Buffer A and then incubated in Buffer B (EDTA 3 mM, EGTA 0.2 mM, DTT 1 mM, Halt protease and phosphatase inhibitor cocktail from Thermo Fisher Scientific) for 30 min on ice. After centrifugation (1,700 rcf, 5 min, 4 °C), the supernatant was collected as the soluble nuclear fraction. The pellet was washed once with Buffer B and resuspended in the same buffer, then sonicated three times for 10 s at 25% amplitude with a Sonics Vibra Cell Ultrasonic processor. This fraction included the chromatin-enriched fraction. Laemmli buffer was added and cell extracts were boiled for 3 min. Western blot analysis and immunoprecipitation Proteins were separated in 8% Tris-Glycine, NuPAGE Novex 3–8% Tris-Acetate, or bolt 4–12% bis tris gels (Invitrogen) according to supplier instructions and then transferred onto polyvinylidene difluoride membranes (GE Healthcare, Fairfield, USA) in CAPS transfer buffer. For subcellular fractionation, equivalent cell number fraction samples were loaded. Saturation of the membrane was achieved by soaking for 1 h in PBS Tween 0.1% containing 5% non-fat milk. The antibodies used for immunodetection were: Actin (MAB 1501, 1:50,000, Merck Millipore, Darmstadt, DE), Cdc6–180.2 (sc-9964, 1:500, Santa Cruz Biotechnology, Dallas, USA), Cdt1 (8064, 1:1,000, Cell Signaling, Danvers, USA), Mcm2 (ab4461, 1:2,000, Abcam), Mcm4-G7 (sc-28317, 1:2,000, Santa Cruz Biotechnology), Mcm5 (ab17967, 1:5,000, Abcam), Mcm7 (sc-22782, 1:1,000, Santa Cruz Biotechnology), Orc2 (M055-3, 1:1,000, MBL, Woburn, USA, or 4736, 1:1,000, Cell Signaling), Orc4 (−2:Santa Cruz-Sc-136331, 1:1,000), Rif1 (A300–569A, 1:1,000, Bethyl, Montgomery, USA), Pol Alpha (ab311777, 1:250, Abcam), Pol Delta (sc-17776, 1:500, Santa Cruz Biotechnology), Tubulin B-5-1-2 (T6074, Sigma Aldrich), DNA-PKcs (ab1832, 1:5,000, Abcam, Cambridge, USA), Chk1 (sc-8408, 1:1,000, Santa Cruz Biotechnology), Phospho-Chk1 (Ser345) (2348, 1:1,000, Cell Signaling), RPA (NA18, 1:1,000, Calbiochem), Phospho-RPA32 (S4/S8) (A300-245A, 1:1,000, Bethyl Laboratories), Chk2 (sc-17748, 1:1,000, Santa Cruz Biotechnology), Phospho-Chk2 (Thr68) (2197, 1:1,000, Cell Signaling), horseradish peroxidase (HRP)-conjugated anti-rabbit and HRP-conjugated anti-mouse (1:10,000, Jackson Immuno Research, West Grove, USA), HRP-conjugated anti-rat (1:5,000). Pol θ-antibodies Pol θ-1 (western blot analysis) and Pol θ-2 (immunoprecipitation experiment) are mouse monoclonal antibodies, affinity purified with protein A ceramic hyperDF (Akta System) (0.1 μg ml −1 ). They were raised against the peptide antigens CSIFRARKRASLDINKEKPG and HDETSSLLPRKESNIVDDNGC, respectively, derived from regions of the central domain of POLQ. Their specificity was checked using an siRNA strategy. For immunoprecipitation experiments, 20 × 10 6 cells were lysed in 1 ml of IP buffer (Tris 50 mM pH8, NaCl 150 mM, EGTA 3 mM, NP40 1%, protease and phosphatase inhibitors, and kept on ice for 30 min. After centrifugation at 13,000 r.p.m. for 10 min at 4 °C, the supernatant was pre-cleared with 40 μl protein A and G (or G only) dynabeads (Invitrogen) for 1 h at 4 °C and then incubated with 8 μg of anti-Orc2-1 (Abcam—ab68348), 5 μg of anti-Orc4 (1: Tranduction Laboratories—H83120, 1:1,000; 2: Santa Cruz-Sc-136331, 1:1,000) or Pol θ-2 antibodies for 150 min and 40 μl of protein A and G (or only G) dynabeads (Invitrogen) was added for two additional hours. Following three washes with the IP buffer, the immunoprecipitated material was resuspended in 60 μl of Laemmli sample buffer, boiled for 3 min and analysed by western blotting. For experiments revealing Pol θ and Orc2 interaction, Pol θ immunoprecipitation was performed as followed: RKO cell pellets were incubated in hypotonic buffer (10 mM Hepes pH 7.9, 1.5 mM MgCl 2 , 10 mM KCl, 0.5 mM DTT, phenylmethylsulphonyl fluoride (PMSF) 0.2 mM) and pelleted by centrifugation at 4,600 r.p.m. for 5 min at 4 °C. They were then resuspended in hypotonic buffer on ice 10 min, homogenized in a glass dounce homogenizer and nuclei were collected by centrifugation at 6,100 r.p.m. for 15 min at 4 °C. Nuclei (volume v) were then resuspended in v/2 low-salt buffer (20 mM Hepes pH 7.9, 25% glycerol, 1.5 mM MgCl 2 , 20 mM KCl, 0.2 mM EDTA, 0.5 mM DTT, PMSF 0.2 mM) and v/2 high-salt buffer (20 mM Hepes pH 7.9, 25% glycerol, 1.5 mM MgCl 2 , 1.2 M KCl, 0.2 mM EDTA, 0.5 mM DTT, PMSF 0.2 mM) was added. They were then extracted for 30 min and pelleted at 14,500 r.p.m. for 25 min at 4 °C. The supernatant (nuclear extract) was then dialysed in dialysis buffer (20 mM Hepes pH 7.9, 20% glycerol, 100 mM KCl, 0.2 mM EDTA, 0.5 mM DTT, PMSF 0.2 mM) for 90 min at 4 °C. Finally, the dialysed nuclear extract was clarified by centrifugation at 14,500 r.p.m. for 20 min at 4 °C, and benzonase (25 U) was then added. Estimation of origin activity by DNA combing Twenty-four hours after transfection of the RKO cell line with control ( CTRL ) or POLQ ( POLQ-1) siRNA, RKO cells were labelled successively with 50 μM IdU (Sigma-Aldrich) for 15 min, 100 μM CldU for 15 min and 3 h 200 μM thymidine. Genomic DNA was prepared in agarose plugs (0.5 × 10 5 cells per plug) and DNA combing was performed as described previously [62] , [63] , except that agarose plugs were melted for 30 min at 65 °C before adding 8 U of β-agarase (New England Biolabs) for overnight digestion at 42 °C. IdU, CldU and single-stranded DNA were detected with mouse anti-BrdU (347580, 1:20, Becton Dickinson) and Alexa 546 Goat anti-Mouse (A11030, 1:50, Molecular Probes), Rat anti-BrdU (Abc117–7513, 1:20, Seralab) and Alexa 488 Goat anti-Rat IgG (A11017, 1:50, Molecular Probes), and Mouse anti-ssDNA (MAB3034, 1:300, Millipore) and Alexa 647 Goat anti-Mouse IgG2a (A21241, 1:50, Molecular Probes), respectively. IODs and Global Instant Fork density were measured as described [63] , [64] . Seventeen and 12 IOD, as well as 126 and 89 Forks were measured for CTRL and Pol θ siRNA cells, respectively. The non-parametric test of Mann–Whitney was applied to compare data sets from control and Pol θ-depleted cells with the use of 12 forks subgroups for the fork density analysis. Neo-synthesized DNA preparation and microarrays RKO cells transfected with POLQ-1 or CTRL siRNA for 24 h, and MRC5-SV cells that stably overexpress Pol θ and its isogenic control cells, were incubated with BrdU (50 μM) for 1 h then collected, washed three times in PBS, fixed in 75% ethanol and stored at −20 °C. Fixed cells were re-suspended first in PBS with RNAse (0.5 mg ml −1 ) and then with propidium iodide (50 μg ml −1 ) followed by an incubation of 30 min at RT. Cells (80,000) were sorted in two fractions, S1 and S2, using INFLUX 500 (Cytopeia BD Biosciences) corresponding to early and late S-phase fractions, respectively. Neo-synthesized DNA was immunoprecipited with BrdU antibodies (Anti-BrdU Pure, BD Biosciences, 347580) as described [65] . To control the quality of enrichment of early and late fractions in S1 and S2, quantitative PCR was performed with CAV2 oligonucleotides (early control) and with bgGRM8 oligonucleotides (late control). Microarray hybridization requires a minimum of 500 ng of DNA and to obtain sufficient specific immunoprecipited DNA, whole-genome amplification was conducted (WGA, Sigma). To be sure that this step did not introduce bias, an after WGA quantitative PCR was performed to confirm the specific enrichment in both the S1 and S2 fractions. After amplification, early and late neo-synthesized DNA were labelled with Cy3 and Cy5 ULS molecules (Genomic DNA Labelling Kit, Agilent) as recommended by the manufacturer. The hybridization was performed according to the manufacturer’s instructions on 4 × 180 K human microarrays (SurePrint G3 Human CGH Microarray Kit, 4 × 180 K, Agilent Technologies, genome reference Hg18) that covers the whole genome with one probe every 13 Kb (11 KB in RefSeq sequences). Microarrays were scanned with an Agilent High-Resolution C Scanner using a resolution of 2 μm and the autofocus option. Feature extraction was performed with the Feature Extraction 9.1 software (Agilent Technologies). For each experiment, the raw data sets were automatically normalized by the Feature extraction software. Analysis was performed with the Agilent Genomic Workbench 5.0 software. The log 2 -ratio timing profiles were smoothed using the Triangular Moving Average option of the Agilent Genomic Workbench 5.0 software with the linear algorithm and 500-kb windows. Identification of replication domains To determine the replication domains in Pol θ-depleted RKO cells and in Pol θ-overexpressing MRC5-SV cells, the algorithms from CGH applications in the Agilent Genomic Workbench 5.0 software were used, particularly the Aberration detection algorithms that define the boundaries and magnitudes of the regions of DNA loss or gain when integrating the Z -score. It finds genomic intervals with an over- or underabundance of probes with log ratios that deviate significantly from baseline with a threshold of 1.8. Results from the Z- score identify regions of enriched probe log ratio change, and can suggest early domains when the log-ratio is positive and late domain when the log-ratio is negative. A comparison was conducted between early and late domains from both cell lines to determine segments where replication timing changes. As mentioned by Hiratani et al . [31] , two major changes can be characterized. The intersection between CTRL siRNA late and POLQ-1 siRNA early intervals will reveal segments that have become earlier by the depletion of Pol θ, and conversely with CTRL siRNA early versus POLQ-1 siRNA late domains, intervals that have become later will be characterized. Similarly, the intersection between MRC5- CTRL late and MRC5-overexpressing Pol θ early intervals will reveal segments that have become earlier by the overexpression of Pol θ, and conversely with MRC5- CTRL early versus MRC5-overexpressing Pol θ late domains, intervals that have become late will be characterized. The intersection was performed with GALAXY tools ( https://main.g2.bx.psu.edu/ [66] ). Line-1 and GC contents The Line-1 element content was extracted with the Profile Annotation tool from GALAXY. For the GC content, two steps were required: (i) determination of the DNA sequence from intervals performed with the Extract Genomic DNA tool; and (ii) calculation of the GC content by the GeeCee EMBOSS tool installed on the GALAXY website. For the Line-1 content, we used the coverage tool from the GALAXY website. G4/GC content The coordinates of the G4 in the human genome (hg 18) were determined by Python script as described in: http://code.google.com/p/bioinformatics-misc/source/browse/trunk/quadparser.py?spec=svn3&r=3 . Next, G4 content was obtained with the coverage tool and normalization with the GC content was performed with the result obtained above. How to cite this article: Fernandez-Vidal, A. et al . A role for DNA polymerase θ in the timing of DNA replication. Nat. Commun. 4:4285 doi: 10.1038/ncomms5285 (2014). Accession codes : The data reported in this paper have been deposited in the Gene Expression Omnibus (GEO), www.ncbi.nlm.nih.gov/geo (accession no. GSE49693 for depleted Polθ experiments and accession number GSE53070 for overexpressed Pol θ experiments).